RNAi-based functional selection identifies novel cell migration determinants dependent on PI3K and AKT pathways Lentiviral short hairpin RNA (shRNA)-mediated genetic screening is a powerful tool for identifying loss-of-function phenotype in mammalian cells. Here, we report the identification of 91 cell migration-regulating genes using unbiased genome-wide functional genetic selection. Individual knockdown or cDNA overexpression of a set of 10 candidates reveals that most of these cell migration determinants are strongly dependent on the PI3K/PTEN/AKT pathway and on their downstream signals, such as FOXO1 and p70S6K1. ALK, one of the cell migration promoting genes, uniquely uses p55γ regulatory subunit of PI3K, rather than more common p85 subunit, to trigger the activation of the PI3K-AKT pathway. Our method enables the rapid and cost-effective genome-wide selection of cell migration regulators. Our results emphasize the importance of the PI3K/PTEN/AKT pathway as a point of convergence for multiple regulators of cell migration. Cell migration is a dynamic process that requires coordinated cytoskeletal regulation and proper polarization, and is governed by the extracellular microenvironment, such as chemokines and growth factors. Cell migration is central to development, wound repair and tissue remodelling, and plays a major role in cancer metastasis [1] , [2] . Cell migration to specific sites of inflammation or infection is also essential for immune system function, with respect to the elimination of foreign or infectious agents [3] . Given the relevance of cell migration in a variety of physiological and pathological conditions, we attempted to identify novel genes that regulate cell migration using the short hairpin RNA (shRNA)-based functional selection of cell migration phenotypes. Lentivirally delivered shRNAs were used to produce stable transcript knockdown in mouse fibroblast cells and to conduct loss of function genetic selections. Genetic screening for genes that regulate cell migration and morphology has been previously performed in various invertebrate model organisms, such as, Drosophila melanogaster and Caenorhabditis elegans [4] , [5] . The development of small interfering RNA (siRNA) and shRNA technology has also made it feasible to perform genetic screening in mammalian cells. siRNAs can be generated in organisms using shRNAs, consisting of a sequence of 21–29 nt, a short loop region, and the reverse complement of the 21–29 nt region [6] . shRNA libraries have been used to perform genetic screens in tissue culture cells for a variety of phenotypes [7] . Recent studies have analysed the closures of scratches in cellular monolayers after growth factor stimulation, using siRNA library targeting kinase and phosphatase genes [8] , [9] . siRNA-based screening was performed to identify regulators of multiple cell adhesion complex formation [10] , and RNAi screening to identify inhibitors of cell migration using SKOV-3 cells (a highly motile ovarian carcinoma cell line) [11] . More recently, new regulators of morphology, cytoskeletal organization and cell migration in human cells have been identified using genome-wide RNAi morphology screening data in D. melanogaster cells [12] . Pooled shRNAs were also used for the genome-wide screen of cell migration regulators [13] , and, in that study, barcode microarray analysis was used to identify enriched shRNAs. Herein, we adopted a selection and sequencing strategy to identify both cell migration-accelerating and -impairing genes using a genome-wide pooled shRNA library. Selection was performed using Boyden chamber assays followed by the separation and enrichment of cells with increased or decreased motility. shRNAs were then retrieved from selected cells and directly identified by half-hairpin barcode sequencing. This selection process resulted in the identification of 91 positive or negative regulators of cell migration; 29 of which genes had not been previously reported as cell migration regulators by RNAi screening. A set of 10 shRNAs was chosen for further validation studies, and these revealed remarkable dependences on the phosphoinositide-3 kinase (PI3K)/phosphatase and tensin homologue (PTEN)/AKT signalling pathway for cell migration acceleration or impairment. Genome-wide functional selection of cell migration regulators To identify novel cell migration-regulating genes, RNAi-based functional selection was performed. After introducing 63,996 pooled lentiviral mouse shRNAs targeting 21,332 genes into NIH3T3 mouse fibroblast cells, the shRNAs that accelerated or impaired baseline motility were selected using the transwell migration assay ( Fig. 1a ). Pooled recombinant lentivirus expressing shRNAs was generated by transfecting HEK293T cells with pHAGE-mir30-RFP -shRNA (targeting the mouse genome) ( Fig. 1b ), pVSV-G , pTat , pPM2 and pRev . NIH3T3 fibroblast cells were infected with the 63,996 pooled lentiviral mouse shRNA library at a multiplicity of infection (m.o.i.) of one [14] , [15] . Two days after infection, shRNA-infected cells were selected with puromycin, placed into the upper compartment of a transwell unit and allowed to migrate through the perforated membrane to the lower compartment. Cells that exhibited accelerated or impaired migration were isolated from lower or upper compartments after 5 or 24 h of incubation, respectively; 5 and 24 h were chosen as optimal incubation times for these purposes ( Supplementary Fig. 1 ). In fact, different cell types and assay conditions were used in the previous migration screens. 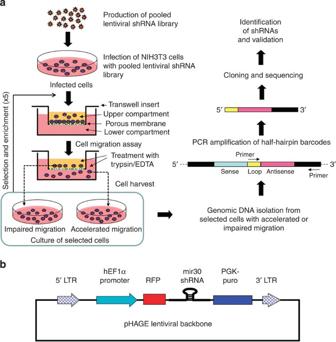Figure 1: Schematic representation of the RNAi-based selection of cell migration regulators. (a) Overview of the selection procedure. The production and infection of genome-wide lentiviral shRNA library are described in Methods. Two days after lentiviral infection, NIH3T3 mouse fibroblast cells were seeded onto transwell inserts and allowed to migrate across the porous membrane at 37 °C for 5 or 24 h, to select cells with an increased or decreased migration phenotype, respectively. Migrated or non-migrated cells were collected by trypsin-EDTA treatment from the lower or upper faces, respectively, of inserts, and reseeded onto transwell culture inserts for a second round of selection (this process was repeated five times). After the final round of selection, shRNAs were retrieved by PCR from selected cells and identified by sequencing. (b) Diagram ofpHAGE-mir30-RFP-shRNA vector. The pooled lentiviral vector contained 63,996 different mir30-based shRNAs targeting 21,332 mouse genes. These discrepancies in the experimental setups may determine the degree of agreement of the current results with published data ( Supplementary Table 1 ). Cells with the desired phenotypes were enriched by repeating the procedure five times. After enrichment, genomic DNA was isolated, and shRNAs integrated into chromosomes were retrieved by PCR amplification, cloned and sequenced. The determined sequences of half-hairpin barcode were used to identify the shRNAs. This selection method identified 91 shRNAs that accelerated or impaired migration ( Tables 1 and 2 ). Sixty-two of the 91 identified target genes have been previously associated with cell migration by RNAi screen [8] , [9] , [10] , [13] , [16] ( Supplementary Tables 2 and 3 ). The remaining 29 target genes had not been previously identified as cell migration regulators by RNAi screen. To determine relationships between cell migration regulators, a signalling network was built by ingenuity pathway analysis (IPA) analysis ( Fig. 2 ). This analysis revealed that the newly identified cell migration regulators were closely linked to various cell movement signalling components ( Fig. 2a ). The 91 cell migration-regulating genes identified were mapped to several major biological functions by IPA analysis; these functions included cell movement and morphology (41%), cellular assembly and organization (21%), cell-to-cell signalling (20%), and protein trafficking and molecular transport (18%) ( Fig. 2b ). Functional sub-networks were also constructed based on the biological functions in which they participate ( Supplementary Fig. 2a–d ). Sub-network topology indicated a close interaction between the newly identified cell migration regulators and various functional components. Direct or indirect protein–protein interactions were also found between the identified regulators and other cell migration signalling components ( Supplementary Fig. 2e ). Several additional targets were identified, not found in the primary selection, which might be predicted to modulate cell migration through network inference; these include CTNNB1, CDK4, MYC, IRS4, EIF3F, KIF5C and so on. In addition, a partial cell migration network was constructed, based on signalling pathways initiated by growth factor/receptor tyrosine kinase, fibronectin/integrin or chemotactic factor/GPCR ( Supplementary Fig. 2f ). Many nodes in the network were candidate genes identified in the current selection. PI3K, PTEN and AKT emerged as convergent points in multiple networks. This result was not surprising, as the PI3K/AKT axis is known to regulate cell migration under diverse conditions. In addition, subcellular localization and disease association of the cell migration-regulating genes were analysed ( Supplementary Fig. 3 and Supplementary Tables 4 and 5 ). The majority of the genes were associated with cancer and neurological diseases. Figure 1: Schematic representation of the RNAi-based selection of cell migration regulators. ( a ) Overview of the selection procedure. The production and infection of genome-wide lentiviral shRNA library are described in Methods. Two days after lentiviral infection, NIH3T3 mouse fibroblast cells were seeded onto transwell inserts and allowed to migrate across the porous membrane at 37 °C for 5 or 24 h, to select cells with an increased or decreased migration phenotype, respectively. Migrated or non-migrated cells were collected by trypsin-EDTA treatment from the lower or upper faces, respectively, of inserts, and reseeded onto transwell culture inserts for a second round of selection (this process was repeated five times). After the final round of selection, shRNAs were retrieved by PCR from selected cells and identified by sequencing. ( b ) Diagram of pHAGE-mir30-RFP -shRNA vector. The pooled lentiviral vector contained 63,996 different mir30-based shRNAs targeting 21,332 mouse genes. Full size image Table 1 List of shRNAs that accelerated cell migration (with targets genes inhibiting cell migration). 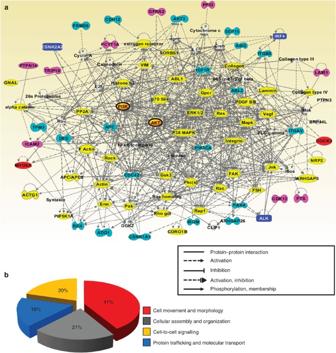Figure 2: Construction of the signalling network of cell migration regulators and their classification based on biological functions. (a) A relevant signalling network was constructed from the 91 cell migration-regulating genes identified by ingenuity pathway analysis (IPA). Newly identified cell migration regulators were linked to various previously reported cell movement signalling components (yellow). Green, cell migration-accelerating genes; blue, cell migration-accelerating genes validated by siRNA; pink, cell migration-impairing genes; red, cell migration-impairing genes validated by siRNA study. PI3K and AKT are highlighted in brown. (b) The biological functions of cell migration regulators were categorized by IPA analysis, which showed 41% were cell movement and morphology related, 21% were cellular assembly and organization related, 20% were cell-to-cell signalling related and 18% were protein trafficking and molecular transport related. Full size table Table 2 List of shRNAs that impaired cell migration (with targets genes promoting cell migration). Full size table Figure 2: Construction of the signalling network of cell migration regulators and their classification based on biological functions. ( a ) A relevant signalling network was constructed from the 91 cell migration-regulating genes identified by ingenuity pathway analysis (IPA). Newly identified cell migration regulators were linked to various previously reported cell movement signalling components (yellow). Green, cell migration-accelerating genes; blue, cell migration-accelerating genes validated by siRNA; pink, cell migration-impairing genes; red, cell migration-impairing genes validated by siRNA study. PI3K and AKT are highlighted in brown. ( b ) The biological functions of cell migration regulators were categorized by IPA analysis, which showed 41% were cell movement and morphology related, 21% were cellular assembly and organization related, 20% were cell-to-cell signalling related and 18% were protein trafficking and molecular transport related. Full size image Validation of selected cell migration regulators Among the 91 shRNAs identified ( Tables 1 and 2 ), 10 were selected for further investigation ( Supplementary Table 6 ). These shRNAs were selected, as little or no evidence linked the corresponding target genes with the regulation of cell migration. shRNA-induced phenotypes were validated using siRNA-mediated knockdown. 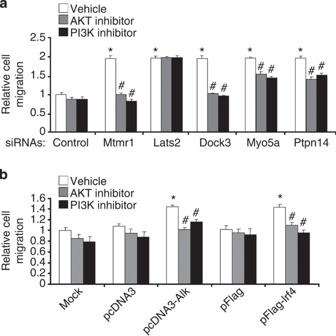Figure 6: Dependences of selected cell migration regulators on the PI3K/AKT pathway. (a) NIH3T3 cells were transiently transfected with control siRNA or siRNAs targetingmtmr1(#5),lats2(#3),dock3(#1),myo5a(#3) orptpn14(#5). After 24 h, wound-healing assay was conducted and cell migration was quantified in the presence or absence of AKT inhibitor (5 μM) or PI3K inhibitor (LY294002; 15 μM). The results shown are means±s.d. (n=3). *P-values of <0.05 indicate significantly different from control siRNA-transfected cells;#P-values of <0.05 indicate significantly different from the corresponding siRNA-transfected cells not treated with inhibitor. (b) Alternatively, NIH3T3 cells were transiently transfected with empty vector (pcDNA3) oralkorirf4expression constructs (pcDNA3-alkorpFlag-irf4) for 24 h. Wound-healing assay was performed to evaluate cell migration in the presence or absence of AKT inhibitor (5 μM) or PI3K inhibitor (LY294002; 15 μM). The results shown are mean±s.d. (n=3). *P-values of <0.05 indicate significantly different frompcDNA3orpFlagempty vector transfected cells;#P-values of <0.05 indicate significantly different from the cells under a similar condition without the inhibitor treatment. To avoid off-target effects, five siRNA duplexes were synthesized for each shRNA candidate identified. Targeting sequences of the siRNAs were distinct from those of the shRNA constructs. The wound-healing assay revealed that transfection with the siRNAs of five migration-accelerating shRNA candidates ( mtmr1 , lats2 , dock3 , myo5a and ptpn14 ) ( Fig. 3a,b ) or with the siRNAs of five migration-impairing shRNA candidates ( csnk2a2 , arid4a , ppp3cc , irf4 and alk ) ( Fig. 3c,d ) increased or decreased, respectively, the motility of NIH3T3 fibroblast cells as compared with control siRNA transfectant. The cell migration-regulating activities of these candidates were also examined using the transwell migration assay, and similar results were obtained ( Fig. 4a,b ). In addition, the cell migration-regulating activities of these candidates were confirmed in L929 mouse fibroblast and mouse embryonic fibroblast (MEF) cells using the transwell migration assay, which indicated that the observed cell migration-regulating effects of the siRNAs were not limited to a single cell line ( Fig. 4c,d ). siRNA-mediated knockdown of the 10 target genes mentioned above was confirmed by RT-PCR ( Fig. 3b,d ), and >50% knockdown was achieved for all siRNAs tested. siRNA-mediated knockdown of the target genes was also confirmed at the protein levels by western blot analysis ( Supplementary Fig. 4a–e ). Furthermore, it should be noted that the cell migration-regulating properties of siRNAs in the wound-healing assay and transwell migration assay were not due to effects on cell proliferation, as determined by MTT assay ( Supplementary Fig. 4f–h ). Validation experiments were extended to other hits identified in the selection and network-derived candidates. Additional 36 hits (20 migration-accelerating shRNAs and 16 migration-impairing shRNAs) and four network-derived candidates ( ctnnb1 , cdk4 , myc and irs4 ) were tested using pooled retroviral shRNAs ( Supplementary Table 7 , Supplementary Fig. 5 and Supplementary Movies 1–3 ). As a result, 71.7% (33/46) of the hits showed cell migration-regulating activity consistent with the primary screen. 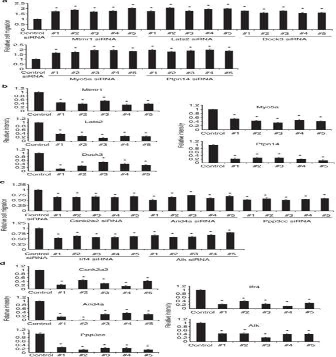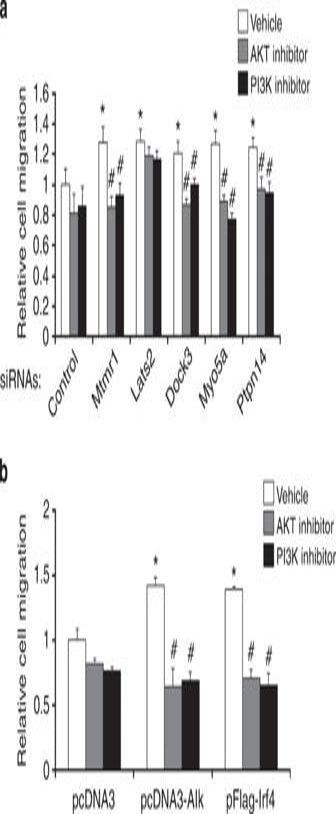Figure 7: Dependence of selected cell migration regulators on the PI3K/AKT pathway determined by three-dimensional cell migration assay. NIH3T3 cells were transiently transfected with either siRNAs targeted formtmr1,lats2,dock3,myo5aandptpn14(a) oralkandirf4expression constructs (pcDNA3-alkorpFlag-irf4) (b). After 24 h of transfection, NIH3T3 fibroblast cells (4 × 104cells/well) were seeded onto the transwell culture inserts and incubated in the presence or absence of either AKT inhibitor (5 μM) or PI3K inhibitor (LY294002; 15 μM) at 37 °C for 6 h. After incubation, non-migrated cells were removed from the upper face of the transwell culture insert. The cells that migrated across the membrane were stained and counted as described in the main text. The results are mean±s.d. (n=3). *P<0.05 represents significantly different from control siRNA-transfected cells;#P<0.05 represents significantly different from the corresponding siRNA-transfected cells without the inhibitor treatment. Among the four network-derived candidates, ctnnb1 and cdk4 shRNAs promoted and inhibited cell migration, respectively, thereby demonstrating 50% validation for the network analysis. Figure 3: Validation of the gene targets found by the RNAi-based functional selection. (a) NIH3T3 fibroblast cells were transiently transfected with control siRNA or one of five siRNAs (#1 to #5) targetingmtmr1,lats2,dock3,myo5aorptpn14. At 24 h after transfection, wound-healing assays were performed to evaluate cell migration. (b) Efficiencies of siRNA-mediated target gene knockdown were confirmed by RT-PCR followed by densitometric analysis. Figure 3: Validation of the gene targets found by the RNAi-based functional selection. ( a ) NIH3T3 fibroblast cells were transiently transfected with control siRNA or one of five siRNAs (#1 to #5) targeting mtmr1 , lats2 , dock3 , myo5a or ptpn14 . 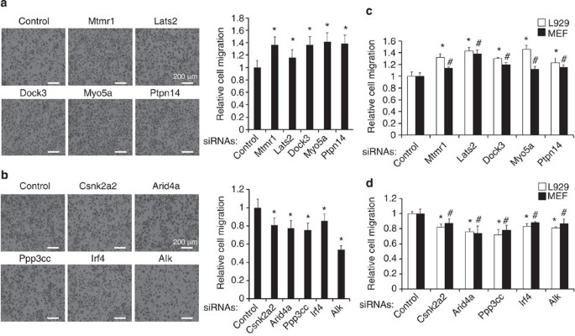At 24 h after transfection, wound-healing assays were performed to evaluate cell migration. ( b ) Efficiencies of siRNA-mediated target gene knockdown were confirmed by RT-PCR followed by densitometric analysis. Figure 4: Validation of shRNA hits by three-dimensional cell migration assay. (a,b) NIH3T3 fibroblast cells were transiently transfected with siRNAs targeting cell migration inhibitors (a) or promoters (b). One siRNA was used for each target:mtmr1(#5),lats2(#3),dock3(#1),myo5a(#3),ptpn14(#5),csnk2a2(#1),arid4a(#1),ppp3cc(#3),irf4(#4) oralk(#3). #1 to #5 indicate the siRNAs used for validation inFig. 3. After 24 h of transfection, NIH3T3 fibroblast cells (4 × 104cells/well) were seeded onto transwell inserts and incubated at 37 °C for 6 h (a; cell migration-accelerating siRNAs) or 9 h (b; cell migration-impairing siRNAs). Non-migrated cells were removed from the upper face of the transwell insert using a cotton swab. Cells that migrated through membranes were stained and counted in five randomly selected fields. The results are representative of three independent experiments (left) or mean±s.d. (n=3) (right). *P<0.05 represents significantly different from control siRNA-transfected NIH3T3 cells. Scale bar, 200 μm. (c,d) L929 fibroblast cells or mouse embryonic fibroblasts (MEFs) were transiently transfected with cell migration-accelerating (c) or impairing (d) siRNAs identified from the screen. After 24 h of transfection, L929 or MEF cells (4 × 104cells/well) were seeded onto the transwell culture inserts and incubated at 37 °C for 6–9 h. After incubation, non-migrated cells were removed from the upper face of the transwell culture insert using a cotton swab. The cells that migrated across the membrane were stained and counted as described in the main text. The results are mean±s.d. (n=3). *P<0.05 represents significantly different from control siRNA-transfected L929 cells.#P<0.05 represents different from control siRNA-transfected MEF cells. Full size image Figure 4: Validation of shRNA hits by three-dimensional cell migration assay. ( a , b ) NIH3T3 fibroblast cells were transiently transfected with siRNAs targeting cell migration inhibitors ( a ) or promoters ( b ). One siRNA was used for each target: mtmr1 (#5), lats2 (#3), dock3 (#1), myo5a (#3), ptpn14 (#5), csnk2a2 (#1), arid4a (#1), ppp3cc (#3), irf4 (#4) or alk (#3). #1 to #5 indicate the siRNAs used for validation in Fig. 3 . After 24 h of transfection, NIH3T3 fibroblast cells (4 × 10 4 cells/well) were seeded onto transwell inserts and incubated at 37 °C for 6 h ( a ; cell migration-accelerating siRNAs) or 9 h ( b ; cell migration-impairing siRNAs). Non-migrated cells were removed from the upper face of the transwell insert using a cotton swab. Cells that migrated through membranes were stained and counted in five randomly selected fields. The results are representative of three independent experiments ( left ) or mean±s.d. ( n =3) ( right ). * P <0.05 represents significantly different from control siRNA-transfected NIH3T3 cells. Scale bar, 200 μm. ( c , d ) L929 fibroblast cells or mouse embryonic fibroblasts (MEFs) were transiently transfected with cell migration-accelerating ( c ) or impairing ( d ) siRNAs identified from the screen. After 24 h of transfection, L929 or MEF cells (4 × 10 4 cells/well) were seeded onto the transwell culture inserts and incubated at 37 °C for 6–9 h. After incubation, non-migrated cells were removed from the upper face of the transwell culture insert using a cotton swab. The cells that migrated across the membrane were stained and counted as described in the main text. The results are mean±s.d. ( n =3). * P <0.05 represents significantly different from control siRNA-transfected L929 cells. # P <0.05 represents different from control siRNA-transfected MEF cells. Full size image Common roles of the PI3K/PTEN/AKT pathways Network analysis of the cell migration regulators identified indicated that the PI3K/PTEN/AKT signalling pathway plays a central role ( Fig. 2 and Supplementary Fig. 2 ). PI3K/PTEN/AKT signalling has been previously associated with cell migration. For example, PI3K/AKT has been reported to enhance actin remodelling, to generate membrane protrusions and to induce cell migration and cell invasion via remodelling of the actin cytoskeleton [17] . PTEN is a lipid phosphatase that dephosphorylates the D3 position of phosphatidylinositol-3,4,5-trisphosphate (PIP3), a second messenger produced by PI3K and that activates AKT [18] , [19] . PTEN is also known to antagonize the cell migration-promoting activity of PI3K. To determine whether the PI3K/PTEN/AKT signalling pathway is involved in the accelerated or impaired migration induced by shRNAs, we first assessed AKT phosphorylation after knocking down dock3 , mtmr1 , ptpn14 , lats2 and myo5a , and after overexpressing alk and irf4 . A knockdown of dock3 , mtmr1 , ptpn14 or myo5a , but not of lats2 , or the overexpression of alk or irf4 induced the phosphorylation of AKT ( Fig. 5a–c ). The overexpression of alk or irf4 in transfectants was confirmed by western blot analysis ( Fig. 5d ). In addition, we used pharmacological inhibitors of PI3K or AKT to evaluate the role of PI3K/AKT signalling in the accelerated or impaired cell migration by shRNAs. siRNA-mediated knockdown was done to upregulate cell migration for cell migration-inhibiting genes, whereas cDNA overexpression was done to upregulate cell migration for cell migration-promoting genes. The accelerated cell migration observed after mtmr1 , dock3 , myo5a or ptpn14 (but not lats2 ) knockdown was significantly attenuated by AKT or PI3K inhibitors in the wound-healing ( Fig. 6a ) and transwell assays ( Fig. 7a ). Similarly, the accelerated cell migration observed for alk or irf4 overexpression was also attenuated by these inhibitors in the wound-healing ( Fig. 6b ) and transwell assays ( Fig. 7b ). Taken together, these results indicate that the cell migration promoters ( csnk2a2 , arid4a , irf4 and alk ) and the inhibitors ( mtmr1 , dock3 , myo5a and ptpn14 ) mediate their effects via the PI3K/AKT pathway. Furthermore, at the concentration used in the current study, the PI3K and AKT inhibitors effectively inhibited downstream signalling pathways and were without effects on cell viability ( Supplementary Fig. 6 ). To gain a better understanding of the role of PI3K/AKT signalling in cell migration following specific gene knockdown, foxo1 and p70s6k1 (downstream components of the AKT pathway) were investigated. The phosphorylation of FOXO1 and p70S6K1 was increased after knockdown of the migration-inhibiting genes dock3 , mtmr1 , ptpn14 and myo5a , and after the upregulation of the migration-promoting genes ( alk and irf4 ) ( Supplementary Fig. 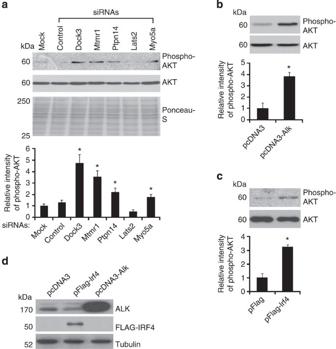7 ). These results support that activation of the PI3K/AKT pathway and downstream events, such as FOXO1 and p70S6K1 phosphorylation, appear to be critically required for diverse cell migration regulators identified by unbiased functional selection. Figure 5: Induction of AKT activation by the selected cell migration regulators. NIH3T3 fibroblast cells were transiently transfected with control siRNA, siRNAs againstdock3(#1),mtmr1(#5),ptpn14(#5),lats2(#3) ormyo5a(#3) (a) or empty vectors (pcDNA3orpFlag),alkorirf4expression constructs (pcDNA3-alkorpFlag-irf4) (b,c). After 48 h, levels of phosphorylated AKT (phospho-AKT at Ser473) or total AKT protein were evaluated by western blot analysis (upper). Ponceau S staining was performed to confirm equal sample loading. The results of densitometric analysis are also shown (lower). The results shown are means±s.d. (n=3); *P-values of <0.05 indicate significantly different from control siRNA- or empty vector-transfected cells. (d) Overexpression of ALK or IRF4 in transfectants was confirmed by western blotting using an anti-ALK or -FLAG-tag antibody. Tubulin was used as the internal control. Figure 5: Induction of AKT activation by the selected cell migration regulators. NIH3T3 fibroblast cells were transiently transfected with control siRNA, siRNAs against dock3 (#1), mtmr1 (#5), ptpn14 (#5), lats2 (#3) or myo5a (#3) ( a ) or empty vectors ( pcDNA3 or pFlag ), alk or irf4 expression constructs ( pcDNA3 - alk or pFlag - irf4 ) ( b , c ). After 48 h, levels of phosphorylated AKT (phospho-AKT at Ser473) or total AKT protein were evaluated by western blot analysis ( upper ). Ponceau S staining was performed to confirm equal sample loading. The results of densitometric analysis are also shown ( lower ). The results shown are means±s.d. ( n =3); * P -values of <0.05 indicate significantly different from control siRNA- or empty vector-transfected cells. ( d ) Overexpression of ALK or IRF4 in transfectants was confirmed by western blotting using an anti-ALK or -FLAG-tag antibody. Tubulin was used as the internal control. Full size image Figure 6: Dependences of selected cell migration regulators on the PI3K/AKT pathway. ( a ) NIH3T3 cells were transiently transfected with control siRNA or siRNAs targeting mtmr1 (#5), lats2 (#3), dock3 (#1), myo5a (#3) or ptpn14 (#5). After 24 h, wound-healing assay was conducted and cell migration was quantified in the presence or absence of AKT inhibitor (5 μM) or PI3K inhibitor (LY294002; 15 μM). The results shown are means±s.d. ( n =3). * P -values of <0.05 indicate significantly different from control siRNA-transfected cells; # P -values of <0.05 indicate significantly different from the corresponding siRNA-transfected cells not treated with inhibitor. ( b ) Alternatively, NIH3T3 cells were transiently transfected with empty vector ( pcDNA3 ) or alk or irf4 expression constructs ( pcDNA3 - alk or pFlag - irf4 ) for 24 h. Wound-healing assay was performed to evaluate cell migration in the presence or absence of AKT inhibitor (5 μM) or PI3K inhibitor (LY294002; 15 μM). The results shown are mean±s.d. ( n =3). * P -values of <0.05 indicate significantly different from pcDNA3 or pFlag empty vector transfected cells; # P -values of <0.05 indicate significantly different from the cells under a similar condition without the inhibitor treatment. Full size image Figure 7: Dependence of selected cell migration regulators on the PI3K/AKT pathway determined by three-dimensional cell migration assay. NIH3T3 cells were transiently transfected with either siRNAs targeted for mtmr1 , lats2 , dock3 , myo5a and ptpn14 ( a ) or alk and irf4 expression constructs ( pcDNA3-alk or pFlag-irf4 ) ( b ). After 24 h of transfection, NIH3T3 fibroblast cells (4 × 10 4 cells/well) were seeded onto the transwell culture inserts and incubated in the presence or absence of either AKT inhibitor (5 μM) or PI3K inhibitor (LY294002; 15 μM) at 37 °C for 6 h. After incubation, non-migrated cells were removed from the upper face of the transwell culture insert. The cells that migrated across the membrane were stained and counted as described in the main text. The results are mean±s.d. ( n =3). * P <0.05 represents significantly different from control siRNA-transfected cells; # P <0.05 represents significantly different from the corresponding siRNA-transfected cells without the inhibitor treatment. Full size image Unique role of p55γ regulatory subunit of PI3K In the next set of experiments, the cell migration-promoting gene alk was subjected to further investigation. Many receptor tyrosine kinases transduce their signals via specific interactions with SH2 domain-containing proteins such as regulatory subunits of PI3K [20] . Therefore, we asked whether the receptor tyrosine kinase alk regulates the PI3K pathway through interaction with regulatory subunits of PI3K. Although anaplastic lymphoma kinase (ALK) physically interacted with both p85α and p55γ regulatory subunits of PI3K ( Fig. 8a,b ), ALK overexpression enhanced phosphorylation of p55γ, but not p85α, subunit ( Fig. 8c ). The ALK-induced phosphorylation of p55γ regulatory subunit of PI3K was accompanied by AKT phosphorylation ( Fig. 8c ) and translocation to the plasma membrane ( Fig. 8d ). GFP-fused AKT-PH domain was used to demonstrate the membrane translocation of AKT [21] . The critical role of p55γ and its phosphorylation in AKT activation and subsequent cell migration was further evaluated by siRNA-mediated knockdown of p55γ ( Fig. 8e,f and Supplementary Fig. 8 ) [22] . p55γ siRNAs decreased ALK-induced AKT phosphorylation and cell migration, further supporting the unique role of p55γ subunit of PI3K in the Alk-promoted cell migration. These results indicate that ALK promotes cell migration by specifically interacting with p55γ subunit of PI3K, rather than more common p85 subunit ( Supplementary Fig. 9a ). 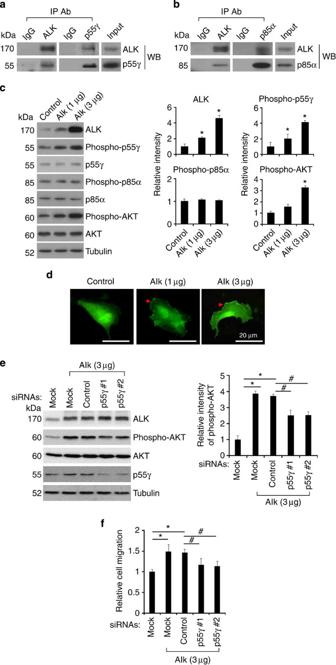Figure 8: Pivotal role of p55γ subunit of PI3K in Alk-mediated cell migration. (a,b) NIH3T3 fibroblast cells were used to reciprocally immunoprecipitate (IP) with anti-ALK and anti-PI3K antibodies as indicated. The precipitated protein was separated on SDS-PAGE and subjected to reciprocal western blot analysis (WB) using each antibody. (c) NIH3T3 fibroblast cells were transiently transfected with control vector (pcDNA3) oralkexpression constructs (pcDNA3-alk). After 48 h, levels of phosphorylated or total ALK, p55γ, p85α and AKT were evaluated by western blotting. Tubulin was used as a loading control. The results of densitometric analysis (right) are mean±s.d. (n=3); *P-values of <0.05 indicate significantly different from control vector-transfected cells. (d) NIH3T3 fibroblast cells on coverslips were transiently transfected with GFP-akt-PH expression construct and control vector (pcDNA3) oralkexpression constructs (pcDNA3-alk). After 36 h, transfected NIH3T3 fibroblast cell images were obtained using fluorescence microscopy to determine the localization of the GFP-AKT-PH. Arrowheads indicate plasma membrane-localized GFP-AKT-PH. Scale bar, 20 μm. (e) ALK-overexpressing NIH3T3 fibroblast cells were transiently transfected with control siRNA or siRNAs againstp55γ. After 48 h, levels of total or phosphorylated AKT, ALK and p55γ were evaluated by western blotting. Tubulin was used as a loading control. The results of phospho-AKT densitometry (right) are means±s.d. (n=3). (f) After 24 h of transfection, NIH3T3 fibroblast cells (4 × 104cells/well) were seeded onto the transwell culture inserts and incubated at 37 °C for 9 h. The cells that migrated across the membrane were stained and counted as described in the main text. The results shown are means±s.d. (n=3); *P-values of <0.05 indicate significantly different from empty vector-transfected cells.#P-values of <0.05 indicate significantly different from control siRNA-transfected cells. Figure 8: Pivotal role of p55γ subunit of PI3K in Alk-mediated cell migration. ( a , b ) NIH3T3 fibroblast cells were used to reciprocally immunoprecipitate (IP) with anti-ALK and anti-PI3K antibodies as indicated. The precipitated protein was separated on SDS-PAGE and subjected to reciprocal western blot analysis (WB) using each antibody. ( c ) NIH3T3 fibroblast cells were transiently transfected with control vector ( pcDNA3 ) or alk expression constructs ( pcDNA3 - alk ). After 48 h, levels of phosphorylated or total ALK, p55γ, p85α and AKT were evaluated by western blotting. Tubulin was used as a loading control. The results of densitometric analysis ( right ) are mean±s.d. ( n =3); * P -values of <0.05 indicate significantly different from control vector-transfected cells. ( d ) NIH3T3 fibroblast cells on coverslips were transiently transfected with GFP- akt -PH expression construct and control vector ( pcDNA3 ) or alk expression constructs ( pcDNA3 - alk ). After 36 h, transfected NIH3T3 fibroblast cell images were obtained using fluorescence microscopy to determine the localization of the GFP-AKT-PH. Arrowheads indicate plasma membrane-localized GFP-AKT-PH. Scale bar, 20 μm. ( e ) ALK-overexpressing NIH3T3 fibroblast cells were transiently transfected with control siRNA or siRNAs against p55γ . After 48 h, levels of total or phosphorylated AKT, ALK and p55γ were evaluated by western blotting. Tubulin was used as a loading control. The results of phospho-AKT densitometry ( right ) are means±s.d. ( n =3). ( f ) After 24 h of transfection, NIH3T3 fibroblast cells (4 × 10 4 cells/well) were seeded onto the transwell culture inserts and incubated at 37 °C for 9 h. The cells that migrated across the membrane were stained and counted as described in the main text. The results shown are means±s.d. ( n =3); * P -values of <0.05 indicate significantly different from empty vector-transfected cells. # P -values of <0.05 indicate significantly different from control siRNA-transfected cells. Full size image We utilized lentivirus-based shRNA libraries targeting the entire mouse genome to enable genome-wide loss-of-function analysis by stable gene knockdown. Broad application of this shRNA library has already been reported in numerous studies on the identification of human disease-related genes [23] , [24] , [25] , [26] , [27] , [28] and genes associated with other phenotypes of interest [29] , [30] , [31] , [32] , [33] . In the current study, we aimed to identify diverse cellular pathways whose knockdowns have positive or negative effects on cell migration phenotypes. Some of the cell migration-regulating genes identified in the present study have well-established links to cellular motility, which validates the selection approach used. We also identified a number of previously uncharacterized cell migration regulators not previously identified by RNAi screening. Importantly, several novel cell migration regulators that were investigated in more detail were found to show marked downstream signalling convergence on the PI3K/PTEN/AKT pathway, which emphasizes the central roles of this pathway in cell migration. Although the RNAi-based functional screening of cell migration regulators has been previously conducted, our approach differs in several ways. First, we performed unbiased genome-scale shRNA selection, rather than screening, as phenotype-driven selection processes reduce false positives and as cells with given phenotypes are separated and enriched several times. The selection method used in the present study is straightforward and cost-effective as compared with array-based RNAi screen. Second, we used cells of fibroblast origin, which have higher baseline motilities than epithelial cells, as this allowed us to select cell migration accelerators and impairers at the same time. In the event, the selection method used identified many migration-promoting and -inhibiting genes not previously reported. Third, we used direct cloning and sequencing of half-hairpin barcodes, rather than microarray analysis, to identify selected shRNAs. This process enabled the unbiased and direct selection of genes contributing to a given phenotype, as microarray-based identification involves statistical evaluation and a degree of ambiguity. In this method, however, it was difficult to assess how representative the selected shRNAs are to the starting shRNA library. Among the functionally diverse 91 hits identified in the primary screen, targets of 13 shRNAs were protein kinases and protein phosphatases. Our results support the validity of the selection methods used and emphasize the critical roles played by protein kinases and phosphatases in cell motility regulation. Some of these kinases and phosphatases were included in our initial validation list, which comprised five migration-accelerating shRNA candidates ( mtmr1 , lats2 , dock3 , myo5a and ptpn14 ) and five migration-impairing shRNA candidates ( csnk2a2 , arid4a , ppp3cc , irf4 and alk ). In later studies, we found that the actions of some of these cell migration regulators, namely, mtmr1 , dock3 , myo5a , ptpn14 , csnk2a2 , alk , irf4 and arid4a (but not lats2 or ppp3cc ), are strongly dependent on the PI3K/PTEN/AKT pathway ( Supplementary Fig. 9b ). Additional validation studies of 36 hits showed 71.7% overall correlation between the results of primary screen and secondary test. Several of the cell migration-regulating genes identified in this study have been previously associated with the PI3K/PTEN/AKT pathway. Casein kinase 2 (CK2 or csnk2 ) is a physiologically relevant PTEN kinase, and CK2-mediated phosphorylation inhibits PTEN function, which in turn increases PIP3 levels, and thus AKT phosphorylation. The expression levels and activities of CK2 subunits have been reported to be increased three- to fivefold in many human cancer and tumour cell lines [34] , [35] , [36] . Protein tyrosine phosphatase non-receptor type 14 ( ptpn14 ) is frequently mutated in a variety of human cancers. However, the cell signalling pathways regulated by Ptpn14 remain largely unknown [37] . In the present study, protein–protein interaction between PTPN14 and PTEN was identified by IPA analysis ( Supplementary Fig. 2e ), which suggests that PTPN14 regulates cell migration by modulating PTEN activity. The physiological role of myotubularin-related protein 1 ( mtmr1 ) has not been clearly determined, although recent studies have shown that mtmr1 is a phosphatase, like myotubularin, and can dephosphorylate both PtdIns3P and PtdIns3,5P2 in vitro [38] , [39] , which suggests its possible involvement in the PI3K/PTEN/AKT pathway. Some of the cell migration regulators identified in this study appear to act independently of the PI3K/PTEN/AKT pathway. Ppp3cc , also known as calcineurin A subunit, is a Ca2+- and calmodulin-dependent serine/threonine protein phosphatase. In a recent study, calcineurin was shown to promote tumour cell invasion via transcriptional factor NFAT in breast cancer metastasis [40] . Lats2 is a serine/threonine protein kinase belonging to the tumour suppressor family, and has been reported to participate in p53 signalling [41] and to be implicated in cell cycle regulation, apoptosis, centrosome duplication and genomic stability [42] , [43] , [44] . Furthermore, our findings suggest that both ppp3cc and lats2 promote or inhibit cell migration, respectively, via a mechanism not involving the PI3K/PTEN/AKT pathway. In the present study, the activations of FOXO1 and p70S6K1 were investigated as signalling events downstream of the PI3K/PTEN/AKT pathway to determine the mechanistic basis of impaired or accelerated cell migration following specific gene knockdown. Forkhead box O (FOXO) proteins, which include FOXO1, FOXO3, FOXO4 and FOXO6, regulate many cancer-related phenotypes by inhibiting nuclear transcription factors. In the previous studies, activation of AKT led to FOXO1 phosphorylation and nuclear exclusion [45] . Furthermore, the nuclear exclusion of FOXO1 abolishes its inhibitory effect on Runx2 activity, and therefore enhances Runx2-mediated gene transcription and the subsequent migration/invasion of cancer cells [46] . In addition, the AKT-mediated phosphorylation of FOXO1 induces its degradation by proteasome [47] , [48] . Consistent with previous findings, we found that the level of FOXO1 was reduced after phosphorylation ( Supplementary Fig. 7 ). In a previous study, mTORC1 and mTORC2 signalling pathways were found to be involved in cytoskeletal rearrangement and cell migration [49] , [50] . In particular, the activations of mTORC1 and p70S6K1 were found to be essential for the migration and invasion of cancer and non-cancer cells via cytoskeletal rearrangement [49] , [51] . In the present study, the phosphorylation of AKT, FOXO1 and p70S6K1 was found to be associated with increased cell migration, which supports the notion that FOXO1 and p70S6K1 are downstream signalling components of PI3K/PTEN/AKT. The PI3K family is categorized into three classes (class I, II, and III) and various subclasses based on their structure, substrate specificity and regulation. The class I PI3K is the best-characterized subfamily present in all cell types. They consist of a p110 catalytic subunit (α, β, γ or δ) and a regulatory subunit (p85α, p85β, p55α, p55γ or p50α) [52] . Regulatory subunits are required to recruit the p110 catalytic subunit to specific cellular locations, thereby regulating its catalytic activity. The different regulatory subunits associate with distinct receptor tyrosine kinases [53] and show the specificity in mediating different PI3K signalling pathways [54] . However, the mechanisms by which these regulatory subunits regulate specific signalling pathways are not fully understood. p55γ, also known as p55PIK, binds the catalytic subunits and modulates PI3K activity in a manner similar to p85α and p85β [54] , [55] . Our data indicate that p55γ was critically involved in the receptor tyrosine kinase Alk-promoted PI3K/AKT activation and cell migration. In the previous reports, p55γ regulatory subunit of PI3K promoted cell cycle progression [56] , DNA synthesis [57] , proliferation and differentiation of leukemia cells [58] , and tumour angiogenesis via regulation of NF-κB signalling or expression of VEGF-A [59] . Furthermore, the protein levels of p55γ increased in colorectal, gastric and ovarian cancers [56] , [59] , [60] . PI3K also plays an important role in the multiple steps of neurite outgrowth during nerve growth factor-stimulated differentiation and in the brain development [61] . ALK was originally identified as an oncogene in human anaplastic large cell lymphoma and neuroblastoma [62] . ALK displays the classical structural features of a receptor tyrosine kinase. In the previous studies, ALK mediated several signal-transduction pathways, including JAK/STAT, RAS/MAPK, PI3K and PLCγ, and modulated various cellular functions, such as proliferation, angiogenesis, metabolism and migration [63] , [64] . An important role of ALK in the development and function of the nervous system has also been reported [65] . Brain expression of ALK changed during mouse [66] or zebrafish [67] embryogenesis, consistent with our results. However, little is known about physiological functions of ALK and its cognate ligands in vertebrate. In this study, for the first time, we have identified the p55γ regulatory subunit of PI3K as a target molecule of ALK during mouse fibroblast cell migration ( Supplementary Fig. 9a ). Physical interaction between ALK and p55γ, ALK-induced phosphorylation of p55γ, and p55γ knockdown studies supported these findings. NIH3T3 cells express three isoforms of AKT. When the involvement of AKT isoforms in the ALK-induced cell migration was examined by knockdown of individual isoforms of akt ( akt1 , akt2 and akt3 ), all three isoforms of AKT were found to play an important role in the ALK-induced migration ( Supplementary Fig. 10 ). Although the critical role of p55γ in the ALK/AKT-induced cell migration has been demonstrated in the current study, it does not necessarily indicate that all the migration-related signalling is mediated via ALK/AKT and p55γ. Also, the phosphorylation of the regulatory subunit p55γ should not be regarded as a definitive indication for increased migration, as the cell migration depends on the relevant downstream PI3K targets and additional regulators. Further studies need to be conducted to better assess the importance of p55γ in cell migration in general. In summary, the selection method used in the present study allowed us to identify a large number of genes that modulated cell migration. Furthermore, many of the cell migration-regulating genes identified have not been previously associated with cell migration. Although the precise regulatory mechanisms responsible for the effects of these cell migration regulators will only be determined by additional studies, the candidate gene list obtained by the current selection process provides an integrated view regarding cell migration. Reagents and cells Specific small-molecule inhibitors, such as Akt inhibitor (1L6-hydroxymethyl-chiro-inositol-2-(R)-2-O-methyl-3-O-octadecyl- sn -glycerocarbon) and PI3K inhibitor (LY294002), were purchased from Calbiochem (La Jolla, CA). Puromycin and mitomycin C were purchased from Sigma-Aldrich (St Louis, MO). All other chemicals, unless otherwise stated, were obtained from Sigma-Aldrich. NIH3T3 mouse fibroblast cells, L929 mouse fibroblast cells and HEK293T human embryonic kidney epithelial cells were maintained in Dulbecco’s modified Eagle’s media (DMEM) supplemented with 10% heat-inactivated fetal bovine serum (FBS) (Invitrogen, Carlsbad, CA), 100 U ml −1 penicillin and 100 μg ml −1 streptomycin (Gibco-BRL, Rockville, MD). Phoenix Ampho cells were cultured in DMEM containing 10% FBS (Lonza, Walkersville, MD), hygromycin B (300 μg ml −1 ) and diphtheria toxin (1 μg ml −1 ) at 37 °C and 5% CO 2 . MEF cell cultures were prepared from 13.5-day-old embryos of Institute for Cancer Research (ICR) mice [68] . Lentivirus production and titration A 63,996 pooled lentiviral shRNA library targeting 21,332 mouse genes was generated by the transient transfection of HEK293T cells with pHAGE-mir30-RFP -shRNA (targeting the mouse genome), pVSV-G , pTat , pPM2 and pRev using LipofectAMINE 2000 (Invitrogen), in accordance with the manufacturer’s instructions. The mir30-based shRNA constructs have been previously described [14] . Cell-free supernatants were collected 2-3 days after transfection and were subsequently used to transduce NIH3T3 cells in the presence of 8 μg ml −1 polybrene. After 24 h, virus-containing supernatants were removed by centrifugation. To optimize conditions for viral infection and to monitor virus titres, NIH3T3 fibroblast cells (1 × 10 6 cells) were seeded onto 100-mm culture plates 18 h before infection and then incubated with 1 ml of red fluorescence protein-carrying lentiviral stock for 6–8 h, in the presence of polybrene (8 μg ml −1 ). Fresh DMEM/10% FBS (2 ml) containing polybrene (8 μg ml −1 ) was then added to the culture and incubation was continued. After another 24 h, cells were removed from plates, and infection efficiencies and viral titres were determined by observing red fluorescence protein under a fluorescence microscope (Olympus BX50; Tokyo). The titre of the viral shRNA library was ~7.23 × 10 6 p.f.u. ml −1 . Selection of cell migration regulators using shRNA library NIH3T3 fibroblast cells were seeded at the density of 1 × 10 6 cells/100-mm culture plate. Three plates of NIH3T3 cells were infected with the lentiviral shRNA library at an m.o.i. of 1 in the presence of polybrene (8 μg ml −1 ) (45 × representation for each shRNA). Two days after infection, cells were puromycin (10 ng ml −1 )-selected for 7 days, detached, seeded onto transwell culture inserts (8-μm pore membrane; Millipore, Billerica, MA) in 24-well plates (~4 × 10 4 cells/transwell culture insert/well) and incubated at 37 °C for either 5 or 24 h. The 5-h time point was used to select migration enhancers and 24 h was used to identify inhibitors of migration. Upper and lower transwell chambers were filled with media containing 0% or 10% FBS, respectively, to induce the directional movement of cells. Infected cells (~3 × 10 6 cells) were divided and placed onto 72 transwell culture inserts. Cells that did or did not migrate were collected by trypsinizing cells adherent to the lower or upper faces of transwell culture inserts, respectively, and then reseeded onto transwell culture inserts. Cells from 72 individual wells were then allowed to re-migrate five times for enrichment purposes. Selected cells from the 72 transwell culture inserts were then combined. To identity the shRNAs integrated into the combined cells, a small amount (50 ng) of genomic DNA separately isolated from migrating or non-migrating cells was subjected to PCR. shRNA segments were amplified using the primer set: forward primer JH353F , TAGTGAAGCCACAGATGTA ; reverse primer BC1R , CCTCCCCTACCCGGTAGA [14] . The resulting PCR fragments (453 bp) were gel-purified, cloned and sequenced [69] ( Fig. 1 ). All clones were sequenced. The sequences of 22–27 nt, corresponding to the half-hairpins of shRNAs, were used to identify shRNAs. Validation of primary hits using retroviral shRNAs Retroviral shRNAs were generated by transient transfection of Phoenix Ampho packaging cells with each shRNA using Lipofectamine 2000 in accordance with the manufacturer’s instructions. Cell-free supernatants were harvested 2–3 days after transfection and subsequently were used to transduce NIH3T3 fibroblast cells in the presence of 8 μg ml −1 polybrene. To optimize conditions of viral infection and to monitor virus titre, a test construct of the retroviral vector carrying GFP ( pFB-hrGFP ) (Stratagene) was used. For infection of NIH3T3 fibroblast cells, cells (1 × 10 5 cells/well) were seeded onto 60-mm culture plates 18 h before infection and incubated with 1 ml of virus stock for 6–8 h in the presence of polybrene (8 μg ml −1 ). Then, 2 ml of fresh DMEM/10% FBS containing polybrene (8 μg ml −1 ) was added to the culture and the incubation was continued. After another 24 h, cells were removed from the plates, and infection efficiency and viral titre were determined by the count of GFP-positive cells using FACS. NIH3T3 fibroblast cells were infected with the retroviral shRNA at an m.o.i. of 1–3. For high-throughput screening, Essen Incucyte and Woundmaker (Essen BioScience, Ann Arbor, MI) were used. In brief, the cell migration algorithm analyzed each image and assigned a well-specific wound mask that corresponded to the initial scratch wound. Scratch wound mask followed migrating cells as they moved into the initial wound, creating a measurement of relative wound density or wound closure. Pathway and network analyses The accession numbers of identified DNAs were exported to IPA (Ingenuity Systems) for network analysis. The statistical significance of each network or list was determined by IPA using Fisher’s Exact test ( P <0.05). IPA was also used to construct networks of protein–protein and other regulatory interactions. For pathway construction, the IPA database used currently available knowledge on genes, proteins, chemicals, normal and disease cellular processes, signalling and cellular functions. Transient transfection with siRNA or cDNA Desalted and preannealed siRNA duplexes were purchased from Genolution Pharmaceuticals (Seoul, Korea). The siRNAs were designed using a proprietary algorithm devised by Genolution Pharmaceuticals. Sequence information for the siRNAs used for validation is given in Supplementary Table 6 . To knockdown specific gene expression, NIH3T3 mouse fibroblast cells were transfected with siRNAs at a final concentration of 10 nM using LipofectAMINE (Invitrogen), according to the manufacturer’s instructions. Cells were harvested 24–48 h after transfection, and the potencies of siRNAs to silence gene expression were measured by RT-PCR or western blot analysis. A control random sequence siRNA was also purchased from Genolution Pharmaceuticals and used as negative control. The full-length cDNAs of mouse alk or irf4 were cloned into the expression vectors pcDNA3 or pFlag , respectively. NIH3T3 fibroblast cells in six-well plates were transiently transfected with 3 μg of alk or irf4 cDNA using LipofectAMINE. The empty vector pcDNA3 or pFlag was used as control for the transient expression of alk or irf4 . One or two days after transfection, cells were used for experiments. The expressions of alk and irf4 mRNAs and proteins in transient transfectants were confirmed by RT-PCR or western blot analysis, respectively. Reverse transcription-PCR Total RNA was extracted from NIH3T3 cells in six-well plates using TRIzol reagent (Invitrogen), according to the manufacturer’s instructions. Reverse transcription was conducted using Superscript II (Invitrogen) and oligo(dT) primer. PCR amplification, using specific primer sets, was carried out at an annealing temperature of 55–60 °C for 20–30 cycles. PCR was performed by using a DNA Engine Tetrad Peltier Thermal Cycler (MJ Research, Waltham, MA). To analyse PCR products, 10 μl of each PCR reaction product was electrophoresed on 1% agarose gel followed by ethidium bromide staining and detection under UV light. β - Actin was used as internal control. The nucleotide sequences of the primers used were based on published cDNA sequences ( Supplementary Table 8 ). Wound-healing assay For the in vitro wound-healing assay, a scratch was created by using a 10-μl pipette tip on confluent cell monolayers in 24-well culture plates, and then DMEM containing 10% FBS, 100 U ml −1 penicillin and 100 μg ml −1 streptomycin was added. Cells were then incubated at 37 °C under 5% CO 2 to enable migration into wounds, which were then observed under a light microscope (Olympus CK2; X100). To rule out confounding effect of cell proliferation, cells were treated with the mitosis inhibitor mitomycin-C at a final concentration of 10 μg ml −1 for 2 h before wounding. Relative cell migration distances were calculated by subtracting final wound widths from initial values [70] . Three non-overlapping fields were selected and examined per well (three wells per experimental group). The results are presented as fold increases in migration distance versus control condition. Three-dimensional cell migration assay Cell migration was also measured using transwell culture inserts (8-μm pore membrane; Millipore), according to the manufacturer’s instructions. In brief, cells were transfected with the siRNAs of migration accelerating or impairing genes. At 24 h after transfection, cells were harvested by trypsinization, resuspended in DMEM and added to upper wells at 4 × 10 4 cells/well. Growth media were placed into base wells, which were separated from top wells by a polycarbonate filter membrane. Cells were incubated at 37 °C for 6 h (for accelerating siRNAs) or 9 h (for impairing siRNAs). Non-migrating cells on the inner sides of transwell culture inserts were then removed with a cotton swab, and migrated cells on the undersides of inserts were fixed with methanol for 10 min and stained with Mayer’s haematoxylin (DakoCytomation, Glostrup, Denmark) for 20 min. Photomicrographs of five random fields were taken (Olympus CK2; X100), and cells were then counted using a NIH image J program (NIH Image; Bethesda, MD). In brief, images were binary thresholded at 50% of the background level, and particles were then converted to a sub-threshold image area with a size >200 pixels, which was determined to be sufficient to identify migrated cells. Numbers of cells were counted and results were analysed statistically. Western blot analysis Cells were lysed in triple-detergent lysis buffer (50 mM Tris-HCl, pH 8.0, 150 mM NaCl, 0.02% sodium azide, 0.1% SDS, 1% NP-40, 0.5% sodium deoxycholate and 1 mM phenylmethylsulfonyl fluoride). Protein concentrations in cell lysates were determined using the Bio-Rad protein assay kit (Bio-Rad, Hercules, CA). Equal amounts of protein were separated by 8 or 12% SDS-PAGE and transferred to Hybond ECL nitrocellulose membranes (Amersham Biosciences, Piscataway, NJ). Membranes were blocked with 5% skim milk and sequentially incubated with primary antibodies (rabbit polyclonal anti-phospho-PI3 kinase p85α (Tyr458)/p55γ (Tyr199) antibody (1:500 dilution; Cell Signaling Technology, Danvers, MA); rabbit polyclonal anti-PI3 kinase p85α antibody (1:1,000 dilution; Cell Signaling Technology); goat polyclonal anti-p55γ antibody (1:500 dilution; Santa Cruz, Santa Cruz, CA); rabbit polyclonal anti-phospho-AKT (Ser473) antibody (1:1,000 dilution; Cell Signaling Technology); rabbit polyclonal anti-AKT antibody (1:1,000 dilution; Cell Signaling Technology); rabbit polyclonal anti-phospho-FOXO1 (Ser256) antibody (1:500 dilution; Cell Signaling Technology); rabbit polyclonal anti-FOXO1 antibody (1:500 dilution; Cell Signaling Technology); rabbit polyclonal anti-phospho-p70S6 kinase (Thr389) antibody (1:1,000 dilution; Cell Signaling Technology); rabbit polyclonal anti-p70S6 kinase antibody (1:1,000 dilution; Cell signaling Technology); monoclonal anti-α-tubulin antibody (1:2,000 dilution; Sigma-Aldrich); rabbit polyclonal anti-MTMR1 antibody (1:500 dilution; Sigma-Aldrich); goat polyclonal anti-PTPN14 antibody (1:500 dilution; Santa Cruz); rabbit polyclonal anti-DOCK3 antibody (1:500 dilution; Abcam, Cambridge, MA); rabbit polyclonal anti-IRF4 antibody (1:500 dilution; Cell Signaling Technology); rabbit polyclonal anti-ALK antibody (1:500 dilution; Novus Biologicals, and HRP-conjugated secondary antibodies (1:10,000 dilution; anti-rabbit-, anti-mouse-, or anti-goat-IgG antibody; Amersham Biosciences), and then detected using an ECL detection kit (Amersham Biosciences). Assessment of cell proliferation and viability by MTT assay NIH3T3 cells in 96-well culture plates were transfected with siRNAs or cDNA constructs and incubated for 24–72 h. At each designated time point after transfection, culture media were removed, MTT (3-[4,5-dimethylthiazol-2-yl]-2,5-diphenyltetrazolium bromide) (0.5 mg ml −1 was added and cells were incubated at 37 °C for 2 h in a CO 2 incubator. After dissolving the insoluble crystals that formed in DMSO, absorbance was measured at 570 nm using a microplate reader (Anthos Labtec Instruments, Wals, Austria). Statistical analysis Results are presented as the means±s.d. of three or more independent experiments, unless stated otherwise. The one-way ANOVA with Dunnett’s multiple-comparison test was used to compare treatments. SPSS version 18.0 K (SPSS, Chicago, IL) was used for the analysis, and P -value differences of <0.05 were considered statistically significant. How to cite this article: Seo, M. et al . RNAi-based functional selection identifies novel cell migration determinants dependent on PI3K and AKT pathways. Nat. Commun. 5:5217 doi: 10.1038/ncomms6217 (2014).